Amorphous nickel hydroxide nanospheres with ultrahigh capacitance and energy density as electrochemical pseudocapacitor materials Among numerous active electrode materials, nickel hydroxide is a promising electrode in electrochemical capacitors. Nickel hydroxide research has thus far focused on the crystalline rather than the amorphous phase, despite the impressive electrochemical properties of the latter, which includes an improved electrochemical efficiency due to disorder. Here we demonstrate high-performance electrochemical supercapacitors prepared from amorphous nickel hydroxide nanospheres synthesized via simple, green electrochemistry. The amorphous nickel hydroxide electrode exhibits high capacitance (2,188 F g −1 ), and the asymmetric pseudocapacitors of the amorphous nickel hydroxide exhibit high capacitance (153 F g −1 ), high energy density (35.7 W h kg −1 at a power density of 490 W kg −1 ) and super-long cycle life (97% and 81% charge retentions after 5,000 and 10,000 cycles, respectively). The integrated electrochemical performance of the amorphous nickel hydroxide is commensurate with crystalline materials in supercapacitors. These findings promote the application of amorphous nanostructures as advanced electrochemical pseudocapacitor materials. Supercapacitors or electrochemical capacitors have attracted considerable interest as energy-storage devices in recent years. Supercapacitors can be classified into two types based on their charge-storage mechanism, electrical double-layer capacitors dominated by electrostatic charge diffusion and accumulation at the interface of the electrode/electrolyte and pseudocapacitors governed by Faradaic reactions at the electrode materials [1] , [2] , [3] . Among numerous active electrode materials, nickel hydroxide (Ni(OH) 2 ) has been recognized as a promising electrode material in electrochemical capacitors [4] , [5] . Almost all of the attention is focused on crystalline Ni(OH) 2 materials mainly because of their flexibility in forming complex three-dimensional (3D) structures and their excellent electrochemical properties in rechargeable alkaline battery applications [4] , [5] , [6] , [7] , [8] , [9] , [10] , [11] , [12] , [13] . Amorphous Ni(OH) 2 materials are usually assessed as unsuitable electrochemical capacitors because of their poor performance [14] . However, the amorphous phase offers a rather unique electrochemical behaviour [15] , [16] , [17] that may be exploitable in certain device applications. In our study, we synthesize amorphous Ni(OH) 2 nanospheres using a simple, low-cost, green-technology electrochemistry technique [18] and then fabricate various supercapacitors from these nanospheres. Our measurements indicate that similar to pseudocapacitors, these nanospheres exhibit excellent electrochemical performance, including high capacitance and energy density and super-long cycle life. Even more, the performance of these amorphous-phase nanospheres in supercapacitors is commensurate with that of its crystalline counterpart [4] , [5] , [6] , [7] , [8] , [9] , [10] , [11] , [12] , [13] , [19] . This discovery promotes the application of amorphous-phase nanomaterials as advanced electrochemical pseudocapacitor materials. Structure and morphology of the amorphous Ni(OH) 2 nanospheres The typical low-magnification scanning electron microscopy (SEM) image ( Fig. 1a ) clearly illustrates the as-synthesized samples composed of many well-defined nanospheres with wrinkled surfaces. The high-magnification SEM image ( Fig. 1b ) reveals that the synthesized nanospheres are approximately 400 nm in diameter with ravine-like surfaces. No crystalline morphology is detected in the bright-field transmission electron microscopy (TEM) image of the sample ( Fig. 1c ). The detailed structure characterizations using high-resolution TEM ( Fig. 1d ) also reveal densely wrinkled surfaces. Thus, we conclude that these nanospheres possess a highly irregular 3D structure. In a corresponding selected-area electron-diffraction pattern (the inset of Fig. 1c ), we observe a broad and diffused halo ring, which indicates an amorphous morphology. In addition, except for the peaks associated with the graphite substrate, no peaks are present in the X-ray diffraction pattern of the as-synthesized sample in Supplementary Fig. S2 , which further confirms the amorphous nature of the sample. 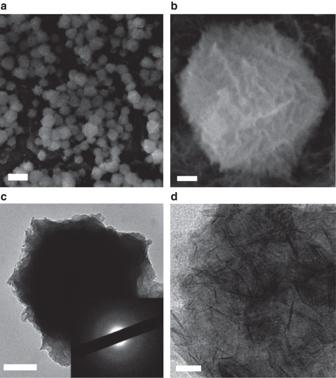Figure 1: Microscopy measurements of amorphous Ni(OH)2samples. (a,b) SEM images of the amorphous Ni(OH)2samples synthesized on graphite electrodes. (c,d) TEM images of the amorphous Ni(OH)2samples (the inset shows the corresponding selected-area electron-diffraction pattern). Scale bars, 1 μm (a), 100 nm (b), 0.2 μm (c) and 20 nm (d). Figure 1: Microscopy measurements of amorphous Ni(OH) 2 samples. ( a , b ) SEM images of the amorphous Ni(OH) 2 samples synthesized on graphite electrodes. ( c , d ) TEM images of the amorphous Ni(OH) 2 samples (the inset shows the corresponding selected-area electron-diffraction pattern). Scale bars, 1 μm ( a ), 100 nm ( b ), 0.2 μm ( c ) and 20 nm ( d ). Full size image X-ray photoelectron spectroscopy (XPS) was used to measure the binding energy, from which we could estimate the various chemical states of bonded elements. Typical spectra of the samples are presented in Fig. 2a . The Ni LMM Auger spectrum contains a single peak whose kinetic energy is at 840.8 eV, which correlates with previously reported data [20] . Two major peaks with binding energies at 857.2 and 874.8 eV correspond to Ni 2p 3/2 and Ni 2p 1/2 , respectively, yielding a spin-energy separation of 17.6 eV characteristic of the Ni(OH) 2 phase, which is in good agreement with a previous report [6] , [7] . In addition, the O 1s spectrum with a strong peak at 532.3 eV is associated with bound hydroxide groups (OH − ) [21] . 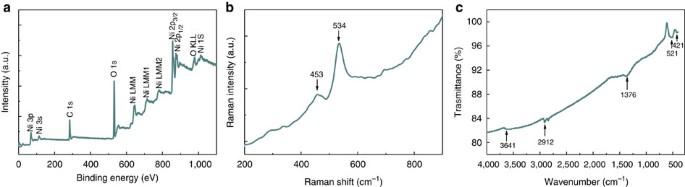Figure 2: Spectroscopy analyses of amorphous Ni(OH)2samples. (a) XPS, (b) Raman and (c) infrared spectra of samples. Figure 2: Spectroscopy analyses of amorphous Ni(OH) 2 samples. ( a ) XPS, ( b ) Raman and ( c ) infrared spectra of samples. Full size image The Raman and infrared spectra of the samples ( Fig. 2b ) exhibit features that are typical of Ni(OH) 2 . In particular, the two broad peaks at 453 and 534 cm −1 ( Fig. 2b ) can be attributed to the symmetric Ni–OH stretching mode [22] , [23] and to vibrations of the Ni–O stretching mode [22] , [23] , [24] and/or to modes associated with structural defects, respectively. The latter are sensitive to crystalline order [24] and defects [23] . The absorption bands are blue-shifted compared with those of the crystalline phase, possibly due to the many defects and disorder within the amorphous phase. Infrared spectroscopy was performed over the range 400–4,000 cm −1 ( Fig. 2c ) to further confirm the XPS and Raman results. Five absorption bands at 421, 521, 1,376, 2,912 and 3,641 cm −1 appear in the spectrum. The two lowest bands at 421 and 521 cm −1 are due to the ν Ni-OH and the δ OH vibrations [23] , [24] . The broad band at 3,641 cm −1 corresponds to the O–H vibration of the hydrogen-bonded hydroxyl groups and intercalated water molecules located in the interlamellar spaces of Ni(OH) 2 (refs 23 , 24 ). The band at 1,376 cm −1 can be attributed to the ν C=O vibration of the absorbed CO 2 molecules, whereas the 2,926 cm −1 band is proposed to be associated with the infrared active vibrations of H 2 O that is absorbed on the sample [6] , [25] . In summary, the SEM, TEM, XPS, infrared and Raman measurements indicate that the as-synthesized samples are amorphous Ni(OH) 2 nanospheres with irregular surface features. Electrochemical characterization of amorphous Ni(OH) 2 nanospheres The capacitive behaviour of an electrode material is generally characterized using current–voltage (CV) curves. 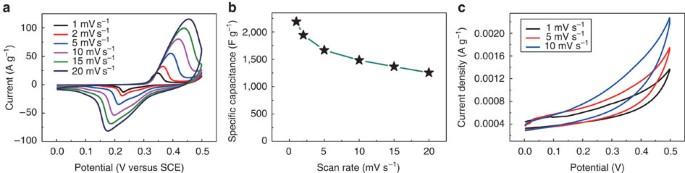Figure 3: Electrochemical characterization of amorphous Ni(OH)2electrode and blank electrode. (a) CV curves of the amorphous Ni(OH)2nanospheres at various scan rates in 1 M KOH. (b) Specific capacitance of the amorphous Ni(OH)2nanospheres as a function of the scan rates based on the CV curves. (c) CV curves of the blank electrode at various scan rates in 1 M KOH. Figure 3a presents typical CV curves of the amorphous Ni(OH) 2 samples in a 1 M KOH electrolyte at various scan rates between 0.0 and 0.5 V. Two strong redox peaks can be observed in each curve. For electric double-layer capacitors, CV curves appear nearly rectangular; however, for Faradaic redox reactions, large redox current peaks are present. Our results thus indicate that the capacitance characteristics are mainly due to Faradaic redox reactions. For the Ni(OH) 2 electrode materials, the surface Faradaic reactions will proceed as [6] Figure 3: Electrochemical characterization of amorphous Ni(OH) 2 electrode and blank electrode. ( a ) CV curves of the amorphous Ni(OH) 2 nanospheres at various scan rates in 1 M KOH. ( b ) Specific capacitance of the amorphous Ni(OH) 2 nanospheres as a function of the scan rates based on the CV curves. ( c ) CV curves of the blank electrode at various scan rates in 1 M KOH. Full size image The anodic and cathodic peaks are observed to be symmetric, suggesting that the reversibility for the as-synthesized amorphous Ni(OH) 2 nanospheres is excellent. These nanospheres are also excellent electron conductors with small equivalent series resistance demonstrated by the minimal change in shape of the CV curves as the scan rate increases from 1 to 20 mV s −1 ; the anodic and cathodic peaks, however, are shifted with increasing scan rate due to the internal resistance of the electrode. The specific capacitance C (F g −1 ), one of the most important parameters for characterizing the electrochemical performance of capacitors, can be calculated from the area under the CV curve [6] , [11] , [25] , [26] , where m is the mass of the electroactive materials in the electrodes (g), v is the potential scan rate (mV s −1 ), V a is the anodic potential (V), V c is the cathodic potential (V), I(V) is the response current density (A) and V is the potential (V). The mass of the as-synthesized Ni(OH) 2 nanospheres was 0.12 mg cm −2 . Therefore, the specific capacitances of the amorphous Ni(OH) 2 samples were calculated to be 2,188, 1,943, 1,667, 1,484, 1,367 and 1,250 F g −1 at scan rates of 1, 2, 5, 10, 15 and 20 mV s −1 , respectively. With increasing scan rate, the specific capacitance decreases gradually ( Fig. 3b ), which can be attributed to electrolytic ions diffusing and migrating into the active materials at low scan rates. At high scan rates, the diffusion effect, limiting the migration of the electrolytic ions, causes some active surface areas to become inaccessible for charge storage. We also observe that the specific capacitance of the amorphous Ni(OH) 2 samples decreases to 1,250 F g −1 as the scan rate increases to 20 mV s −1 , representing only a 43% decrease compared with the specific capacitance at a scan rate of 1 mV s −1 . This result indicates the excellent capacitive behaviour and high-rate capability of the amorphous phase. Note that the measured capacitance of the amorphous Ni(OH) 2 nanospheres is much higher than that of α- and β-Ni(OH) 2 materials such as α-Ni(OH) 2 /graphene (1,735 F g −1 ) [6] and β-Ni(OH) 2 nanoplates/graphite (1,335 F g −1 ) [4] . To eliminate the exaggerated capacitance of Ni(OH) 2 as a current collector in the electrochemical measurement, CV curves of a blank electrode, a pure graphite substrate not containing any deposited amorphous Ni(OH) 2 , were measured under similar conditions ( Fig. 3c ). These curves reveal that the current is much lower than for the Ni(OH) 2 electrode, indicating that the current arising from the blank electrode can be neglected. Moreover, the specific capacitance of the blank electrode calculated from the CV curve at a scan rate 1 mV s −1 is 0.192 F g −1 , which is much lower than that of the Ni(OH) 2 electrode, confirming the CV results. Note that the mass of the blank graphite is 0.180 g cm −2 in this case. To further evaluate the electrochemical properties and estimate the stable potential windows of the as-synthesized amorphous Ni(OH) 2 nanospheres, galvanostatic charging and discharging of the amorphous Ni(OH) 2 nanospheres in 1 M KOH solution were performed using a Pt counter electrode and a saturated calomel reference electrode. The charge–discharge curves ( Fig. 4a ) at different current densities (20–70 A g −1 ) between 0.0 and 0.5 V display slight nonlinearities that are very distinct from those of typical pure double-layer capacitors. This result, corroborating previous reports [4] , [8] , [9] , [11] , indicates the occurrence of Faradaic reactions in the amorphous Ni(OH) 2 . In other words, the shape of the discharge curves is representative of pseudo-capacitance, which substantiates the CV curve results. 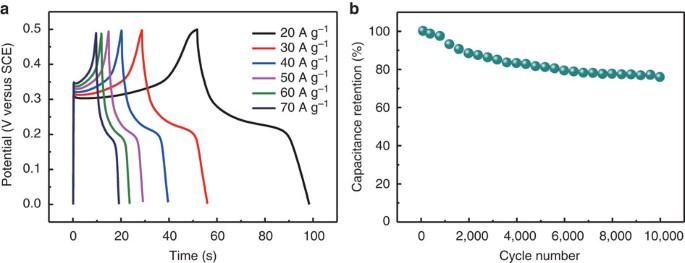Figure 4: Electrochemical stability of amorphous Ni(OH)2samples. (a) Charge–discharge curves of amorphous Ni(OH)2nanospheres at various current densities (ranging from 20 to 70 A g−1). (b) Cycle performance of amorphous Ni(OH)2samples measured at a scan rate of 100 mV s−1for 10,000 cycles. Figure 4: Electrochemical stability of amorphous Ni(OH) 2 samples. ( a ) Charge–discharge curves of amorphous Ni(OH) 2 nanospheres at various current densities (ranging from 20 to 70 A g −1 ). ( b ) Cycle performance of amorphous Ni(OH) 2 samples measured at a scan rate of 100 mV s −1 for 10,000 cycles. Full size image The specific capacitance of the electrode can be calculated from the discharge curve according to (F g −1 ) (ref. 27 ). Here I is the discharge current (A), is the discharge time (s), m is the mass of the active material in the electrode (g) and Δ V is the potential change during discharge (V). The specific capacitances obtained were 1,868, 1,626, 1,544, 1,430, 1,404 and 1,330 F g −1 at current densities of 20, 30, 40, 50, 60 and 70 A g −1 , respectively. Clearly, the specific capacitance gradually decreases with increasing current density. Over this current density range, the specific capacitance decreases to 72% of its initial value. Moreover, these results are similar to those calculated from the CV curves ( Fig. 3 ), confirming the ultrahigh capacitance of the amorphous Ni(OH) 2 nanospheres. Good cycling stability is another important characteristic for high-performance supercapacitors. Figure 4b reveals the cycle performance of the amorphous Ni(OH) 2 samples measured at a scan rate of 100 mV s −1 for 10,000 cycles. Afterward, the capacitance was 76% of the initial capacitance, indicating excellent long-term stability of the amorphous Ni(OH) 2 nanospheres electrode. The nanospheres lost only ~3% of their initial capacitance after 1,000 cycles. Thus, these results reveal the ultrahigh specific capacitance and remarkable rate capability of the amorphous Ni(OH) 2 nanomaterials for high-performance electrochemical pseudocapacitors. Electrochemical characterizations of the asymmetric capacitors To evaluate the capacitive performance of the Ni(OH) 2 /graphite electrode in a full-cell setup, an amorphous Ni(OH) 2 –active carbon (AC)-based asymmetric capacitor was fabricated in our study. The electrochemical performances of the individual Ni(OH) 2 /graphite electrode and AC/graphite electrode are demonstrated in Supplementary Figs S3 and S4 . The specific capacitance of Ni(OH) 2 and the AC electrode are 1,578 and 177 F g −1 , respectively, which were calculated from the CV curves at scan rates of 5 mV s −1 . The total mass of the active materials on the anode was 0.14 mg cm −2 , and that on the cathode was 0.80 mg cm −2 ; these values are similar to the ideal mass ratio of 0.177 (see Supplementary Methods ). 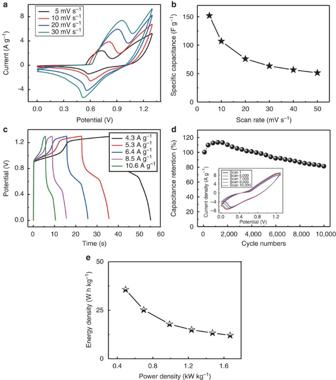Figure 5: Electrochemical characterization of asymmetric capacitor. (a) CV curves of the amorphous Ni(OH)2–AC-based asymmetric capacitor at various scan rates in 1 M KOH. (b) Specific capacitance of the asymmetric capacitor as a function of scan rate based on the CV curves. (c) Charge–discharge curves of the capacitor at various current densities (ranging from 4.3 to 10.6 A g−1). (d) Cycle performance of the asymmetric capacitor measured at a scan rate of 50 mV s−1for 10,000 cycles. (e) Power and energy density of the amorphous Ni(OH)2supercapacitors. The inset presents the CV curves of the asymmetric supercapacitor. Figure 5a presents typical CV curves for the Ni(OH) 2 –AC-based asymmetric capacitor in a 1 M KOH electrolyte at various scan rates between 0.0 and 1.3 V. The two strong redox peaks in each curve indicate the pseudo-capacitive property of the supercapacitor due to Faradaic redox reactions. Moreover, the cell voltage of the asymmetric capacitor increases to 1.3 V. Based on the total mass of the active materials of the two electrodes, Fig. 5b indicates the calculated specific capacitances of the asymmetric cell at various scan rates. It is clear that a specific capacitance of 153 F g −1 is obtained at a scan rate of 5 mV s −1 . The specific capacitance of the device is limited by that of the AC-negative electrode (approximately 175 F g −1 ). Thus, it is very likely that the device capacitance can be further increased by improving the capacitance of the negative electrode. To further evaluate the electrochemical properties and estimate the stable potential windows of the as-fabricated amorphous Ni(OH) 2 –AC-based asymmetric capacitor, galvanostatic charging and discharging of the asymmetric capacitor were performed. Figure 5c presents the charge–discharge curves at various current densities (4.3–10.6 A g −1 ). These curves display slight nonlinearities between 0 and 1.3 V, which confirms the CV results. Figure 5d reveals the cycle performance of the Ni(OH) 2 –AC-based asymmetric capacitor measured at a scan rate of 50 mV s −1 for 10,000 cycles. A total capacitance loss of only 19% is observed after the cell underwent 10,000 cycles, which indicates the excellent long-term stability of the asymmetric capacitor. It is significant that the capacitance retains 97% of its initial capacitance after 5,000 cycles. These results thus demonstrate the high specific capacitance and remarkable rate capability of the amorphous Ni(OH) 2 nanomaterials for high-performance electrochemical pseudocapacitors. The energy density, , and power density, (W g −1 ), are two important parameters that characterize the electrochemical performance of an electrochemical capacitor [6] , [27] , where U 0 is the potential at the end of charge (V) and t is the discharge time (s). Figure 5e presents a Ragone plot, which relates the energy density to the power density of the asymmetric capacitor. The energy density of the supercapacitors decreases from 35.7 to 12.6 W h kg −1 as the power density increases from 0.49 to 1.67 kW kg −1 . Noticeably, we obtained an energy density of 35.7 W h kg −1 at a power density of 490 W kg −1 . Figure 5: Electrochemical characterization of asymmetric capacitor. ( a ) CV curves of the amorphous Ni(OH) 2 –AC-based asymmetric capacitor at various scan rates in 1 M KOH. ( b ) Specific capacitance of the asymmetric capacitor as a function of scan rate based on the CV curves. ( c ) Charge–discharge curves of the capacitor at various current densities (ranging from 4.3 to 10.6 A g −1 ). ( d ) Cycle performance of the asymmetric capacitor measured at a scan rate of 50 mV s −1 for 10,000 cycles. ( e ) Power and energy density of the amorphous Ni(OH) 2 supercapacitors. The inset presents the CV curves of the asymmetric supercapacitor. Full size image Accordingly, we demonstrate for the first time that asymmetric pseudocapacitors prepared from amorphous Ni(OH) 2 nanospheres exhibit good electrochemical performance. In this work, a specific capacitance of 153 F g −1 was obtained at a scan rate of 5 mV s −1 , the energy density for the device was as high as 35.7 W h kg −1 at a power density of 490 W kg −1 , and after 5,000 cycles, the capacitance was 97% of the initial capacitance. For crystalline Ni(OH) 2 materials [6] , a specific capacitance of 125 F g −1 was observed at a scan rate of 5 mV s −1 , the energy density for the device was 45 W h kg −1 at a power density of 500 W kg −1 and the capacitance achieved 94.3% retention after 3,000 cycles. Therefore, we can conclude that the integrated electrochemical performance of the amorphous Ni(OH) 2 nanospheres in supercapacitors is comparable with that of crystalline Ni(OH) 2 materials. Therefore, the application of amorphous Ni(OH) 2 nanospheres as advanced positive electrode materials in capacitors was confirmed for the first time in this study, and the electrochemical performance of the amorphous Ni(OH) 2 –AC-based asymmetric capacitor is commensurate with that of the crystalline Ni (OH) 2 -based asymmetric capacitor [6] , [12] , [28] , [29] , [30] . Considering that the electrochemical performance of Ni(OH) 2 materials largely depends on their surface microstructure and electronic conductivity, we suggest three factors that contribute to the amorphous Ni(OH) 2 nanospheres exhibiting superior electrochemical performance. First, the surface of the as-synthesized amorphous Ni(OH) 2 nanospheres is very clean. The highly pure de-ionized water, used as the electrolyte instead of electrolytic solutions with higher electrical conductivity, provides a chemically clean reaction environment without any chemical additives that ensures production of highly pure and clean surfaces. The clean surface can enable the amorphous Ni(OH) 2 nanospheres to effectively interact with electrolytes. Second, the irregular surfaces of these nanospheres offer large surface areas compared with smooth nanospheres, which increases contact between the electrolytes and electrode materials. As observed in Fig. 1b , the surface of the Ni(OH) 2 nanoparticles possesses a 3D nanostructure, that is, these surfaces are ravine-like, which provides an extremely large surface compared with the smooth surface of crystalline Ni(OH) 2 , thus promoting the electrical conductivity of the electrodes [7] , [8] , [9] . The third factor relates to the amorphous nature of the structures. According to previous work [31] , the disorder in Ni(OH) 2 can greatly improve electrochemical efficiency; indeed, a low-crystalline or amorphous-phase material has the potential to exhibit excellent electrochemical performance because of its high structural disorder. In addition, the amorphous Ni(OH) 2 nanospheres in our samples are directly self-assembled on the surface of the graphite electrode. This self-assembly not only maintains structural continuity but also results in good electrical contact between the nanospheres and the electrode, which is indispensable for good electrochemical performance. In summary, we have synthesized high-purity amorphous Ni(OH) 2 nanospheres using a simple and green electrochemical process. We demonstrated that these nanospheres possess excellent electrochemical performance and that they are suitable as advanced electrode materials for pseudosupercapacitors with high specific capacitance, energy density and power density, as well as a super-long cycle life. The integrated electrochemical performance of these supercapacitors is comparable to that of crystalline Ni(OH) 2 materials. These findings promote new opportunities for amorphous Ni(OH) 2 materials as high-performance supercapacitors and other energy-storage devices. Synthesis of amorphous Ni(OH) 2 nanospheres The amorphous Ni(OH) 2 nanospheres were synthesized using a unique electrochemistry technique that is simple, green and low cost [18] . Two parallel flakes from cleaned graphite were used as the cathode and anode, both with a working area of approximately 1.0 × 1.0 cm 2 . Both electrodes were inserted in a quartz chamber with a separation of approximately 5.0 cm. A target of 99.99% pure nickel, with a diameter of 25.0 mm, was fixed at the center of the chamber floor and immersed in high-purity de-ionized water (18.2 MΩ cm −1 ) without any chemical additives ( Supplementary Fig. S1 ). The technique was performed in constant potential mode with voltage 75 V. Characterization of amorphous Ni(OH) 2 SEM (Quanta 400F) and TEM (JEM-2010HR) were employed to identify the morphology and structure of the as-synthesized samples. To understand the surface information of the as-synthesized samples, XPS (ESCALab250) was conducted to analyse the composition of the sample surface. In addition, infrared and Raman spectra of the samples were obtained to confirm the XPS analysis results. Infrared spectroscopy was performed on a Fourier transformation infrared spectrometer coupled with an infrared microscope (EQUINOX 55) in the range of 400−4,000 cm −1 , and the Raman spectra were obtained using a laser micro-Raman spectrometer (Renishaw inVia) employing an argon-ion laser with an incident wavelength of 514.5 nm. The mass of the as-synthesized amorphous Ni(OH) 2 was measured using inductively coupled plasma-atomic emission spectrometry (TJA, IRIS-DUO-HR). The as-synthesized samples deposited on the graphite electrode were first soaked in a nitric acid solution (10%) for 48 h to ensure that Ni(OH) 2 had completely reacted with the nitric acid. We then measured the gravimetric nickel using the inductively coupled plasma method. Electrochemical characterization of single electrodes and pseudocapacitors The electrochemical measurements were conducted in a three-electrode electrochemical cell with a Pt counter electrode and a saturated calomel reference electrode in a 1 M KOH solution. The graphite electrode upon which as-synthesized amorphous Ni(OH) 2 materials were deposited was used as the working electrode. Cyclic voltammetry measurements were obtained using an electrochemical workstation in the scan range of 0–0.5 V. A graphite sheet (current collector) upon which the as-synthesized amorphous Ni(OH) 2 materials were deposited was used as the positive electrode, and AC was used as the negative positive electrode and was prepared according to the following steps. The mixture containing 80 wt% AC, 10 wt% carbon black and 10 wt% polyvinylidene fluoride was well mixed and dissolved with N -methyl kelpyrrolidide solution and then pressed onto a graphite sheet (current collector). Finally, the electrode was dried at 55 °C for 24 h. The mass of the electrodes were measured using a XP2U Ultra-microbalance ( d =0.1 μg). How to cite this article: Li, H. B. et al . Amorphous nickel hydroxide nanospheres with ultrahigh capacitance and energy density as electrochemical pseudocapacitor materials. Nat. Commun. 4:1894 doi: 10.1038/ncomms2932 (2013).